Singular localization of sodium channel β4 subunit in unmyelinated fibres and its role in the striatum Voltage-gated Na + channel β-subunits are multifunctional molecules that modulate Na + channel activity and regulate cell adhesion, migration and neurite outgrowth. β-subunits including β4 are known to be highly concentrated in the nodes of Ranvier and axon initial segments in myelinated axons. Here we show diffuse β4 localization in striatal projection fibres using transgenic mice that express fluorescent protein in those fibres. These axons are unmyelinated, forming large, inhibitory fibre bundles. Furthermore, we report β4 dimer expression in the mouse brain, with high levels of β4 dimers in the striatal projection fascicles, suggesting a specific role of β4 in those fibres. Scn4b -deficient mice show a resurgent Na + current reduction, decreased repetitive firing frequency in medium spiny neurons and increased failure rates of inhibitory postsynaptic currents evoked with repetitive stimulation, indicating an in vivo channel regulatory role of β4 in the striatum. Voltage-gated Na + channels (VGSCs) are a large, multimeric complex that consists of a pore-forming α-subunit and one or more auxiliary β-subunits [1] . Four different VGSC β-subunits (β1-β4), encoded by genes Scn1b - Scn4b , are expressed in the nervous system [1] , [2] . VGSC β-subunits are multifunctional molecules that modulate Na + current kinetics and regulate channel cell surface expression and neurite outgrowth [3] , [4] , [5] . On the basis of structural and amino-acid homologies, VGSC β-subunits belong to the immunoglobulin superfamily of cell adhesion molecules (IgCAMs) [6] . Thus, a growing hypothesis is that VGSC β-subunits play a crucial role in both modulating action potential firing and cell-adhesion-related activities [2] . β4 is similar to the β2 subunit (35% identity) and contains an extracellular Ig-like domain [7] that interacts with the α-subunit through a cysteine residue. This interaction is required for β4 recruitment at the nodes of Ranvier [8] . β4 is associated with resurgent Na + current ( I NaR ) [9] , [10] —a transient voltage-dependent influx of Na + ions that occurs during repolarization of the membrane after action potentials [11] . C-terminal peptides of β4 may act as a blocking protein in the open Na + channel, inducing I NaR in Purkinje cells [10] . Furthermore, knockdown of Scn4b in cerebellar granule cells reduces I NaR [9] . We have been studying the role of β4 in the pathogenesis of Huntington disease (HD) and found that it is expressed mainly in striatum. In HD transgenic mice, β4 expression is reduced in the early phase of the disease in neurons that express mutant huntingtin (mHtt) [12] . We also found that overexpression of β4 induced neurite outgrowth in neuroblastoma cells and increased spine density in hippocampal cultured neurons [12] , [13] , suggesting a function in cell adhesion as seen for other β-subunits. Regarding the localization of β4, it was recently reported that β4 is enriched in axon initial segments (AIS) and nodes of Ranvier of diverse neuronal types in the brain [8] . However, functional and localization studies have not been conclusive for striatal neurons, which show the highest expression of β4 in the nervous system. In this study, we examine the localization of β4 in striatum and other parts of the brain. In cerebellum and spinal cord, β4 is localized in AIS and nodes of Ranvier as are other β-subunits. In striatal projection axons, however, β4 is diffusely distributed. We further report that the axons of striatal projection neurons form large, unmyelinated inhibitory fibre bundles, which is an intriguing finding as very little is known about the distribution and importance of unmyelinated fibres in the central nervous system. We further show that β4-deficient mice exhibit a reduction of I NaR , disruption of repetitive firing and increased failure rates in medium spiny neurons (MSNs) in the striatum, suggesting that β4 serves as a physiological channel modulator in MSNs. Unique β4 distribution in striatal projection axons It is well known that VGSCs are highly concentrated at the nodes of Ranvier and AIS in myelinated nerve fibres [1] . To examine whether this is true for β4, we first labelled brain sections of wild-type (WT) mice with an antibody specific to the mouse β4 C-terminal peptide (anti-mSCN4B-C) [14] . Dotted β4 immunoreactivity was observed in cerebellar white matter and cervical spinal cord ( Fig. 1a,b ), whereas diffuse β4 staining was observed in long and large axon bundles of basal ganglia ( Fig. 1c ). Next, we performed double staining with anti-SCN4B-C and anti-Kv1.2, a protein of the juxtaparanodal region. As Kv1.2 is also expressed in cerebellar basket cell axon terminals, which project to Purkinje cell AIS [15] , we also used anti-Kv1.2 to detect Purkinje cell AIS. β4 proteins were clustered at the nodes of Ranvier in cerebellar white matter and spinal cord ( Fig. 2a ) and at Purkinje cell AIS ( Fig. 2b ). β1 and Nav1.6, which are VGSC subunits (β and α, respectively), were also localized in the same regions ( Fig. 2a,b ). 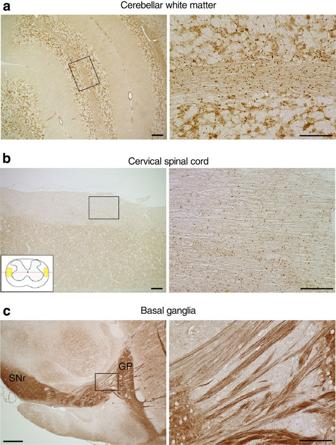Figure 1: β4 distribution in the mouse brain. β4 expression in the 16-week-old mouse brain. Cerebellar white matter (a), lateral funiculus of cervical spinal cord (b) and basal ganglia (c) were stained with anti-SCN4B-C. Right panels show higher magnification of boxed area in left panels. Dissected part of cervical spinal cord is illustrated inside box in (b); longitudinal sections were cut from the red dotted line and the yellow boxed area was observed after immunostaining. The boxed area was also examined in the immunofluorescent studies ofFig. 2(a). Scale bars, 100 μm (a,b, left panels;c, right panel); 50 μm (a,b, right panels); 500 μm (c, left panel). GP, globus pallidus; SNr, substantia nigra pars reticulata. Figure 1: β4 distribution in the mouse brain. β4 expression in the 16-week-old mouse brain. Cerebellar white matter ( a ), lateral funiculus of cervical spinal cord ( b ) and basal ganglia ( c ) were stained with anti-SCN4B-C. Right panels show higher magnification of boxed area in left panels. Dissected part of cervical spinal cord is illustrated inside box in ( b ); longitudinal sections were cut from the red dotted line and the yellow boxed area was observed after immunostaining. The boxed area was also examined in the immunofluorescent studies of Fig. 2 ( a ). Scale bars, 100 μm ( a , b , left panels; c , right panel); 50 μm ( a , b , right panels); 500 μm ( c , left panel). GP, globus pallidus; SNr, substantia nigra pars reticulata. 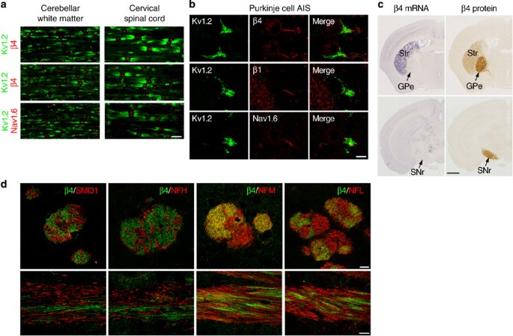Figure 2: Characterization of β4-expressing axons in the mouse brain. (a,b) 17-week-old mouse brain sections were stained with anti-Kv1.2 (green), anti-mSCN4B-C (top panels, red), anti-mSCN1B-C (middle panels, red), anti-Nav1.6 (bottom panels, red). Observed area is described inFig. 1a,b. (c) Distributions of β4 mRNA and β4 protein in the coronal sections of the 12-week-old mouse brain. β4 mRNA is expressed mainly in striatum (Str) and strong β4 immunoreactivity was observed in the external globus pallidus (GPe) and substantia nigra pars reticulata (SNr). (d) Coronal (upper panels) and sagittal (lower panels) sections of 16-week-old mouse striatum were stained with anti-mSCN4B-C (green), anti-SMI31 (red), anti-NFH (red), anti-NFM (red) and anti-NFL (red). Scale bars, 10 μm (a,b,d); 1 mm (c). Full size image Figure 2: Characterization of β4-expressing axons in the mouse brain. ( a , b ) 17-week-old mouse brain sections were stained with anti-Kv1.2 (green), anti-mSCN4B-C (top panels, red), anti-mSCN1B-C (middle panels, red), anti-Nav1.6 (bottom panels, red). Observed area is described in Fig. 1a,b . ( c ) Distributions of β4 mRNA and β4 protein in the coronal sections of the 12-week-old mouse brain. β4 mRNA is expressed mainly in striatum (Str) and strong β4 immunoreactivity was observed in the external globus pallidus (GPe) and substantia nigra pars reticulata (SNr). ( d ) Coronal (upper panels) and sagittal (lower panels) sections of 16-week-old mouse striatum were stained with anti-mSCN4B-C (green), anti-SMI31 (red), anti-NFH (red), anti-NFM (red) and anti-NFL (red). Scale bars, 10 μm ( a , b , d ); 1 mm ( c ). Full size image When we observed β4 distributions macroscopically with in situ hybridization and immunohistochemistry, consistent with our previous report [12] , neurons expressing β4 mRNA were mainly localized in the striatum, but the strongest β4 immunoreactivity was observed in external globus pallidus (GPe) and substantia nigra pars reticulata (SNr) ( Figs 1c and 2c ). A similar observation was previously reported in human striatum [12] . β4 protein seems to be distributed diffusely in axons of striatal projection neurons, which is different from the dotted distribution seen in white matter of the cerebellum and spinal cord ( Fig. 1 ). β4 is enriched in the axons of striatal projection neurons We expected β4 to localize on the axons of striatal projection neurons, based on anti-mSCN4B-C immunoreactivity. In the higher eukaryotes, neurofilaments are the major intermediate filaments in axons. There are three types of neurofilament subunits: heavy (NFH), medium (NFM) and light (NFL) [16] , [17] . To confirm our assumption that β4 is localized along the axons of striatal projection neurons, we first performed double staining with anti-mSCN4B-C and SMI31, which recognizes phosphorylated NFH. Unexpectedly, the β4-positive fibres in the striatum were not labelled with SMI31 ( Fig. 2d ). Another NFH antibody also showed segregated staining from β4-positive fibres ( Fig. 2d ). Immunostaining signals of NFM and NFL in the fascicles showed faint co-localization with anti-SCN4B-C ( Fig. 2d ), suggesting that β4-positive fibres cannot be defined by conventional axonal markers that recognize major cytoskeletal components. Next, to visualize the axons of striatal projection neurons, and to find direct evidence that β4 is expressed in those axons, we generated transgenic mice with the fluorescent marker Venus [18] under the control of the 9-kb Scn4b promoter ( Scn4b-Venus , Fig. 3a ). We found native Venus fluorescence mainly in the striatum ( Fig. 3b ), and Venus co-localized with endogenous β4 mRNA ( Fig. 3c ) and DARPP-32, which is a marker of MSNs ( Fig. 3d ), indicating that β4 was expressed in striatal MSNs. Venus protein must therefore be transported from cell bodies to the processes in this transgenic mouse brain. Immunostaining of sagittal brain sections of Scn4b-Venus using anti-GFP and anti-mSCN4B-C showed that β4-positive fibres completely co-localized with Venus-positive fibres, which projected to globus pallidus (GP) and SNr ( Fig. 3e,f ), suggesting that the fibres are certainly the axons of striatal projection neurons. On the basis of anatomical projection patterns and biochemical differences, MSNs form two pathways. The dopamine D1 receptor (D1R)-positive MSNs project to the medial GP and SNr (direct pathway), whereas dopamine D2 receptor (D2R)-positive MSNs project to the lateral GP (indirect pathway) and co-express enkephalin (PPE encoded by Penk ) [19] . To further confirm that β4 was expressed in the axons of striatopallidal projection neurons, we used PPE-GFP transgenic mice [20] . Anti-GFP can detect the axons of striatopallidal projection neurons and endogenous β4 was co-expressed along those axons ( Fig. 3g,h ). Thus, our results confirmed that β4 is strongly expressed in both axons of direct and indirect pathways. To reveal the positional relation with the axons of nigrostriatal neurons, which are afferent inputs arising from the neurons of substantia nigra pars compacta (SNc), we labelled the axons of nigrostriatal neurons with an anti-tyrosine hydroxylase (TH) antibody, which is a marker of dopamine neurons in SNc. TH-positive axons did not overlap with β4-positive axons in the striatum and SN ( Supplementary Fig. 1 ), where β4-positive axons converge into pars reticulata. 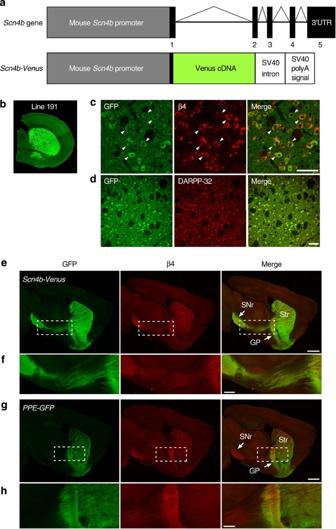Figure 3: β4 is strongly expressed in axon bundles of the striatal projection neuron. (a) Schematic representation of theScn4b-promoter Venus expression cassette. Venus is expressed under the control of the 9-kbScn4b-promoter. (b) Native Venus fluorescence was observed in striatum of line 191Scn4b-Venustransgenic mice. (c) Coronal striatal section of the 8-week-oldScn4b-Venustransgenic mouse was stained by anti-GFP (green) and β4 mRNA (red). Arrows show some of the double-labeled neurons. (d) Coronal striatal sections of 12-week-oldScn4b-Venusmouse were stained with anti-GFP (green) to define β4-positive cells and anti-DARPP-32 (red) to label MSNs. (e–h) 100-μm-thick sagittal brain sections of the 17-weeks-oldScn4b-Venustransgenic mouse (e,f) and the 31-weeks-oldPPE-GFPtransgenic mouse (g,h) were stained with anti-GFP (green) and anti-mSCN4B-C (red). (f,h) Higher magnification of the boxed areas ineandg, respectively. Scale bars, 50 μm (c,d); 1 mm (e,g); 300 μm (f,h). GP, globus pallidus; SNr, substantia nigra pars reticulata; Str, striatum. Figure 3: β4 is strongly expressed in axon bundles of the striatal projection neuron. ( a ) Schematic representation of the Scn4b -promoter Venus expression cassette. Venus is expressed under the control of the 9-kb Scn4b -promoter. ( b ) Native Venus fluorescence was observed in striatum of line 191 Scn4b-Venus transgenic mice. ( c ) Coronal striatal section of the 8-week-old Scn4b-Venus transgenic mouse was stained by anti-GFP (green) and β4 mRNA (red). Arrows show some of the double-labeled neurons. ( d ) Coronal striatal sections of 12-week-old Scn4b-Venus mouse were stained with anti-GFP (green) to define β4-positive cells and anti-DARPP-32 (red) to label MSNs. ( e – h ) 100-μm-thick sagittal brain sections of the 17-weeks-old Scn4b-Venus transgenic mouse ( e , f ) and the 31-weeks-old PPE-GFP transgenic mouse ( g , h ) were stained with anti-GFP (green) and anti-mSCN4B-C (red). ( f , h ) Higher magnification of the boxed areas in e and g , respectively. Scale bars, 50 μm ( c , d ); 1 mm ( e , g ); 300 μm ( f , h ). GP, globus pallidus; SNr, substantia nigra pars reticulata; Str, striatum. Full size image β4-expressing striatal projection axons are unmyelinated Na + channel α and β subunits are highly recruited in the nodes of Ranvier and AIS in myelinated axons. However, we found diffuse, non-focal β4 distribution along the axons of striatal projection neurons, raising the question of whether striatal projection axons could be unmyelinated (that is, lacking nodes of Ranvier). We used Scn4b-Venus mice to investigate this question. Venus co-distributed with endogenous β4 in striatal axons, which were segregated from NFH-positive axons ( Fig. 4a ). To detect the nodes of Ranvier, sagittal Scn4b-Venus striatal sections were stained with anti-Nav1.6 (ref. 21 ) (nodal protein) and anti-Caspr (paranodal protein). Nodes of Ranvier were identified almost exclusively on NFH-positive axons, but not on Venus-positive axons ( Figs 4b,c and 5a,b ), suggesting that β4 expressing striatal projection axons could be unmyelinated. To further confirm this, we performed immunostaining with β4 and MBP, a major constituent of the myelin sheath, and we found the segregation of those stainings ( Figs 4d and 5c–e ). For direct evidence that β4-expressing striatal projection axons are unmyelinated, we performed EM and immunoEM analysis. The fascicles of striatal projection fibres in the striatum and SN were composed of a large number of unmyelinated axons ( Supplementary Fig. 2 ), and the unmyelinated axons were labelled by anti-mSCN4B-C ( Fig. 4e ). β4 immunoreactivity tended to concentrate at the edges of unmyelinated axons ( Fig. 4e , right panel). In addition, to determine the α-subunit that is coexpressed with β4 in striatal projection fibres, we performed immunostaining with antibodies to β4 and Nav1.2, another well-known α-subunit in the central nervous system (CNS) [22] , [23] . Nav1.2 was diffusely distributed in the striatal axons and its immunoreactivity co-localized with β4 ( Fig. 4f ). Futhermore, to confirm whether Nav1.2-bearing fibres are unmyelinated, we performed immunostaining with anti-Nav1.2 and anti-Caspr; Nav1.2 was not co-localized with Caspr ( Fig. 4g ). These results suggest that Nav 1.2 is a major α-subunit of unmyelinated striatal projection fibres. 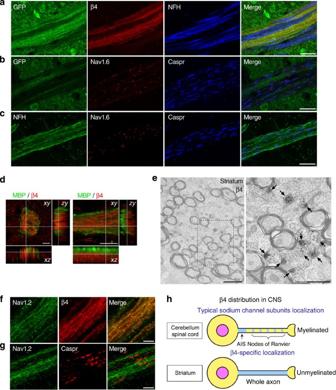Figure 4: β4-expressing striatal projection axons are unmyelinated. (a–c) Sagittal striatal sections of 12-week-oldScn4b-Venusmice were stained with the following sets of antibodies: (a) anti-GFP (green) to detect Venus-positive fibres, anti-mSCN4B-C (red), anti-NFH (blue); (b) anti-GFP (green), anti-Nav1.6 (red), anti-Caspr (blue); (c) anti-NFH (green), anti-Nav1.6 (red), anti-Caspr (blue). (d) Z-stack confocal immunofluorescent images of the fascicles in 15-week-old mouse striatum (left panel, coronal section; right panel, sagittal section), which were stained with anti-MBP (green) and anti-mSCN4B-C (red). Side views show thexzandzyplanes of the fascicles. (e) Immuno EM analysis using anti-SCN4B-C in striatal projection fibres. Right panel shows higher magnification of the boxed area in left panel. Arrows indicate β4-labelled axons. (f,g) Sagittal sections of the striatal fascicles in 17-week-old mice were stained with anti-Nav1.2 (green) and anti-mSCN4B-C (red) (f), anti-Nav1.2 (green) and anti-Caspr (red) (g). (h) Schematic representation of the β4 distributions in myelinated (cerebellum, spinal cord) and unmyelinated axons (striatum). Scale bars, 20 μm (a–d); 1 μm (e, left panel); 0.5 μm (e, right panel); 5 μm (f,g). Figure 4: β4-expressing striatal projection axons are unmyelinated. ( a – c ) Sagittal striatal sections of 12-week-old Scn4b-Venus mice were stained with the following sets of antibodies: ( a ) anti-GFP (green) to detect Venus-positive fibres, anti-mSCN4B-C (red), anti-NFH (blue); ( b ) anti-GFP (green), anti-Nav1.6 (red), anti-Caspr (blue); ( c ) anti-NFH (green), anti-Nav1.6 (red), anti-Caspr (blue). ( d ) Z-stack confocal immunofluorescent images of the fascicles in 15-week-old mouse striatum (left panel, coronal section; right panel, sagittal section), which were stained with anti-MBP (green) and anti-mSCN4B-C (red). Side views show the xz and zy planes of the fascicles. ( e ) Immuno EM analysis using anti-SCN4B-C in striatal projection fibres. Right panel shows higher magnification of the boxed area in left panel. Arrows indicate β4-labelled axons. ( f , g ) Sagittal sections of the striatal fascicles in 17-week-old mice were stained with anti-Nav1.2 (green) and anti-mSCN4B-C (red) ( f ), anti-Nav1.2 (green) and anti-Caspr (red) ( g ). ( h ) Schematic representation of the β4 distributions in myelinated (cerebellum, spinal cord) and unmyelinated axons (striatum). Scale bars, 20 μm ( a – d ); 1 μm ( e , left panel); 0.5 μm ( e , right panel); 5 μm ( f , g ). 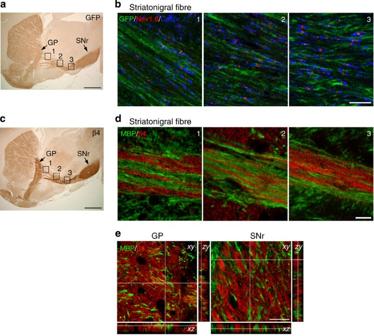Figure 5: Striatonigral fibres show the features of unmyelinated axons along the fibres. (a) Sagittal brain section of 12-week-oldScn4b-Venusmouse stained with anti-GFP to observe Venus-positive β4 expressing axons. Boxed areas are the approximate examined regions of immunofluorescence results in (b). (b) Sagittal brain sections of 12-week-oldScn4b-Venusmouse stained with anti-GFP (green), anti-Nav1.6 (red) and anti-Caspr (blue). (c) Sagittal brain section of 12-week-old mouse stained with anti-mSCN4B-C. Boxed areas are the approximate examined regions of immunofluorescence results in (d). (d,e) Sagittal brain sections of 15- to 17-week-old mice stained with anti-MBP (green) and anti-mSCN4B-C (red). (e) Z-stack confocal immunofluorescence images of GP and SNr. Side views are examined thexzandzyplanes. Scale bar, 1 mm (a,c); 10 μm (b,d); 20 μm (e). GP, globus pallidus; SNr, substantia nigra pars reticulata. Full size image Figure 5: Striatonigral fibres show the features of unmyelinated axons along the fibres. ( a ) Sagittal brain section of 12-week-old Scn4b-Venus mouse stained with anti-GFP to observe Venus-positive β4 expressing axons. Boxed areas are the approximate examined regions of immunofluorescence results in ( b ). ( b ) Sagittal brain sections of 12-week-old Scn4b-Venus mouse stained with anti-GFP (green), anti-Nav1.6 (red) and anti-Caspr (blue). ( c ) Sagittal brain section of 12-week-old mouse stained with anti-mSCN4B-C. Boxed areas are the approximate examined regions of immunofluorescence results in ( d ). ( d , e ) Sagittal brain sections of 15- to 17-week-old mice stained with anti-MBP (green) and anti-mSCN4B-C (red). ( e ) Z-stack confocal immunofluorescence images of GP and SNr. Side views are examined the xz and zy planes. Scale bar, 1 mm ( a , c ); 10 μm ( b , d ); 20 μm ( e ). GP, globus pallidus; SNr, substantia nigra pars reticulata. Full size image Taken together, our results demonstrate that β4-expressing striatal projection axons are unmyelinated. We identified two β4 distribution patterns as follows: in myelinated axons (cerebellum and spinal cord), β4 is recruited to the nodes of Ranvier and AIS, whereas in unmyelinated axons (striatum), β4 is diffusely distributed along the axons ( Fig. 4h ). Establishing a β4-deficient mouse In the CNS, β4 is most highly expressed in the striatum, although the role of β4 protein in the striatum remains unclear. To address this, we generated Scn4b -null mice with or without mCherry-V5-His and neomycin-resistant gene cassettes, which are described as Scn4b −/−(mc) and Scn4b −/− mice, respectively ( Fig. 6a ). Immunoblotting of whole-brain lysate using polyclonal anti-mSCN4B-C and monoclonal anti-hSCN4B-C (7D7F10) ( Supplementary Fig. 3 ) revealed depletion of β4 expression in both Scn4b −/−(mc) and Scn4b −/− mice ( Supplementary Fig. 4a ). In situ hybridization and immunohistochemistry showed that β4 mRNA and β4 protein expression were lost in the striatum of Scn4b −/− mice ( Supplementary Fig. 4b ). 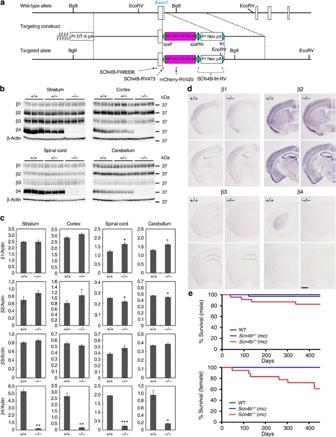Figure 6: Generation and characterization ofScn4b-null mice. (a) Diagram of the targeting strategy to ablateScn4b. Homologous recombination of the targeting construct at theScn4bgene locus resulted in the targeted allele in which the last coding region of exon1 is replaced by mCherry-V5-His and neomycin-resistant gene cassettes. The targeting construct includes LoxP sites (green triangles) that flank mCherry-V5-His cassette and FRT sites (blue triangles) that flank neomycin-resistant gene cassette. The mCherry-V5-His cassette and neomycin-resistant gene cassette were removed by crossbreeding with aCAG-Credeleter mouse and aCAG-FLPedeleter mouse, respectively. The regions of genotyping primers are shown as red lines. (b) Western blot analysis of sodium channel β-subunits. Membrane fractions (20 μg) of the striatum, cortex, spinal cord and cerebellum from 33-week-old WT (+/+), heterozygous (+/−) and homozygous (−/−)Scn4b(mc)mutant mice were immunoblotted using antibodies specific to β-subunits. β-Actin was used as a loading control. (c) Expression levels of β1-4 were quantified. Data are presented as mean±s.e.m. (n=3 for each genotype). *P<0.05, **P<0.01, ***P<0.001, unpaired Student’st-test for β1-3; unpairedttest with Welch’s correction for β4. (d)In situhybridization using cRNA probes of β subunits in WT (+/+) andScn4b−/−(mc)(−/−) mouse brains. Scale bar, 1 mm. (e) Kaplan–Meier survival curves showed sudden unexpected death of male (upper panel) and female (lower panel)Scn4b(mc)mutant mice (male,n=17 for WT;n=34 forScn4b+/−(mc);n=23 forScn4b−/−(mc). female,n=20 for WT;n=14 forScn4b+/−(mc);n=18 forScn4b−/−(mc)).P=0.0231 (male) andP=0.0005 (female), log-rank test. Figure 6: Generation and characterization of Scn4b -null mice. ( a ) Diagram of the targeting strategy to ablate Scn4b . Homologous recombination of the targeting construct at the Scn4b gene locus resulted in the targeted allele in which the last coding region of exon1 is replaced by mCherry-V5-His and neomycin-resistant gene cassettes. The targeting construct includes LoxP sites (green triangles) that flank mCherry-V5-His cassette and FRT sites (blue triangles) that flank neomycin-resistant gene cassette. The mCherry-V5-His cassette and neomycin-resistant gene cassette were removed by crossbreeding with a CAG-Cre deleter mouse and a CAG-FLPe deleter mouse, respectively. The regions of genotyping primers are shown as red lines. ( b ) Western blot analysis of sodium channel β-subunits. Membrane fractions (20 μg) of the striatum, cortex, spinal cord and cerebellum from 33-week-old WT (+/+), heterozygous (+/−) and homozygous (−/−) Scn4b (mc) mutant mice were immunoblotted using antibodies specific to β-subunits. β-Actin was used as a loading control. ( c ) Expression levels of β1-4 were quantified. Data are presented as mean±s.e.m. ( n =3 for each genotype). * P <0.05, ** P <0.01, *** P <0.001, unpaired Student’s t -test for β1-3; unpaired t test with Welch’s correction for β4. ( d ) In situ hybridization using cRNA probes of β subunits in WT (+/+) and Scn4b −/−(mc) (−/−) mouse brains. Scale bar, 1 mm. ( e ) Kaplan–Meier survival curves showed sudden unexpected death of male (upper panel) and female (lower panel) Scn4b (mc) mutant mice (male, n =17 for WT; n =34 for Scn4b +/−(mc) ; n =23 for Scn4b −/−(mc) . female, n =20 for WT; n =14 for Scn4b +/−(mc) ; n =18 for Scn4b −/−(mc) ). P =0.0231 (male) and P =0.0005 (female), log-rank test. Full size image As Na + channels comprise a pore-forming α-subunit and two auxiliary β-subunits, it is possible that another paired β-subunit may compensate for the loss of β4 expression. Western blot analysis using antibodies specific to β-subunits showed that β1 protein levels of Scn4b −/−(mc) were slightly upregulated in the spinal cord and cerebellum, but not in the striatum and cortex ( Fig. 6b,c ). β2 levels of Scn4b −/−(mc) mice were slightly lower in the spinal cord and cerebellum, and β3 levels were not altered in Scn4b −/−(mc) mice. These results suggest that only β1 shows compensatory upregulation in a region-specific manner. Furthermore, we examined whether compensatory localization changes occurred in the brains of Scn4b -null mice, using in situ hybridization of β-subunits. No localization changes were seen in the brains of Scn4b −/−(mc) mice ( Fig. 6d ). Scn4b −/− mice showed sudden unexpected death without apparent abnormality such as seizure ( Fig. 6e ). We observed a subtle tremor-like phenotype in the Scn4b -null mice while holding them. To measure this objectively, we used an accelerometer and found a high-frequency (approximately 20–40 Hz) tremor-like movement in 12-week-old Scn4b − / − mice ( Supplementary Fig. 4c,d ), indicating that loss of β4 induced the tremor-like phenotype. Effect of Scn4b ablation on striatal projection fibres β-subunits are members of the IgCAM family and participate in cell adhesion-related activities through their extracellular domain [2] . β1 and β2 interact in a trans -homophilic manner, and it leads to aggregation of cultured cells and ankyrin recruitment to sites of cell–cell contact [24] , suggesting that homophilic dimer formation could have a role in cell adhesion. Thus, in addition to modulating Na + channel activity, β4 potentially serves as a CAM through its extracellular domain. However, β subunits are cleaved by β- and γ-secretase family proteins [14] and the extracellular domain could be released. Thus, we first confirmed the existence of the extracellular domain of β4 in striatal projection fibres. Immunofluorescence results showed that an antibody specific to the extracellular domain of β4 (anti-mSCN4B-EC) completely co-localized with 7D7F10, an antibody that recognizes the C terminus of β4, in striatal projection fibres ( Fig. 7a and Supplementary Fig. 3 ). This result indicates the existence of an extracellular domain of β4 in striatal projection fibres. Next we performed western blot analysis in an undenatured condition to examine the homophilic interaction of β4. To visualize and dissect striatonigral fibres, we used Scn4b-Venus mice. In the undenatured condition, we found significantly increased dimer formation of β4 in striatonigral fibres compared with other brain regions ( Fig. 7b,c ), suggesting that homophilic β4 interaction might occur between unmyelinated striatal projection axons. Furthermore, the result raised the possibility that the homophilic interaction of β4 seems to play a role in fasciculation and pathfinding of striatal projection fibres. To examine the role of β4 in striatal projection fibres, we observed organization of the fascicles of striatal projection neurons in Scn4b −/− mice by EM. In addition, we performed anti-GFP staining to observe the pathfinding of striatal projection fibres in Scn4b −/−(mc) -Venus mice. However, there were no obvious changes evident in the EM analysis of Scn4b −/− mice ( Fig. 7d ) and anti-GFP staining of striatal projection fibres in Scn4b −/−(mc) -Venus mice ( Fig. 7e ). 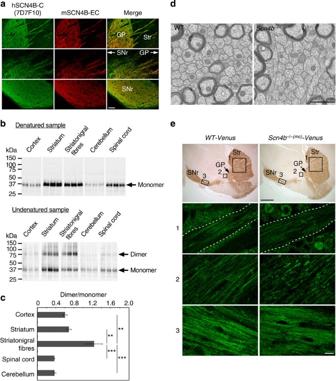Figure 7: Fasciculation of the unmyelinated axons in the striatum is preserved inScn4b−/−mice. (a) Striatonigral fibres of sagittal brain sections of 12-week-old mice were stained with anti-hSCN4B-C (7D7F10) (green) and anti-mSCN4B-EC antiserum (red). (b) Denatured and undenatured brain lysates (20 μg) prepared from the cortex, striatum, striatonigral fibres, cerebellum and spinal cord of 12- to 17-week-oldScn4b-Venusmice were immunoblotted with anti-mSCN4B-C. (c) Ratio of β4 dimer to β4 monomer levels was calculated. Data are presented as mean±s.e.m. (n=3). **P<0.01, ***P<0.001, one-way ANOVA followed by Tukey’spost hoctest. (d) Electron micrographs of cross-sectioned striatal projection fibres in the striatum of 40-week-old WT andScn4b−/−mice. (e) Immunostaining of sagittal brain sections from 12-week-oldWT-VenusandScn4b−/−(mc)-Venusmice with anti-GFP. Top panels are macro view of sagittal brain sections. Boxed areas are the approximate examined regions of immunofluorescence results of the lower panels (1–3). The dotted lines in panel 1 are the outline of the examined axon fascicle. Scale bars, 100 μm (a); 1 μm (d); 1 mm, (e, top panels); 10 μm (e, bottom 1–3 panels). GP, globus pallidus; SNr, substantia nigra pars reticulata; Str, striatum. Figure 7: Fasciculation of the unmyelinated axons in the striatum is preserved in Scn4b −/− mice. ( a ) Striatonigral fibres of sagittal brain sections of 12-week-old mice were stained with anti-hSCN4B-C (7D7F10) (green) and anti-mSCN4B-EC antiserum (red). ( b ) Denatured and undenatured brain lysates (20 μg) prepared from the cortex, striatum, striatonigral fibres, cerebellum and spinal cord of 12- to 17-week-old Scn4b-Venus mice were immunoblotted with anti-mSCN4B-C. ( c ) Ratio of β4 dimer to β4 monomer levels was calculated. Data are presented as mean±s.e.m. ( n =3). ** P <0.01, *** P <0.001, one-way ANOVA followed by Tukey’s post hoc test. ( d ) Electron micrographs of cross-sectioned striatal projection fibres in the striatum of 40-week-old WT and Scn4b −/− mice. ( e ) Immunostaining of sagittal brain sections from 12-week-old WT-Venus and Scn4b −/−(mc) -Venus mice with anti-GFP. Top panels are macro view of sagittal brain sections. Boxed areas are the approximate examined regions of immunofluorescence results of the lower panels (1–3). The dotted lines in panel 1 are the outline of the examined axon fascicle. Scale bars, 100 μm ( a ); 1 μm ( d ); 1 mm, ( e , top panels); 10 μm ( e , bottom 1–3 panels). GP, globus pallidus; SNr, substantia nigra pars reticulata; Str, striatum. Full size image Effect of Scn4b loss on channel function in the striatum To investigate whether β4 indeed regulates I NaR in vivo , we performed electrophysiological analysis of MSNs from the striatum. Medium-sized cells (~10 μm in diameter) isolated from the striatal regions were used for whole-cell voltage clamp recordings of Na + currents ( Fig. 8a ). Most of them were considered to be the projection neurons of the striatum, MSNs, because the other medium-sized GABAergic interneurons such as parvalbumin-containing fast-spiking (FS) neurons and somatostatin/nitric oxide synthase-containing low-threshold spike (LTS) neurons comprise only a small percentage of the striatal neuron population. 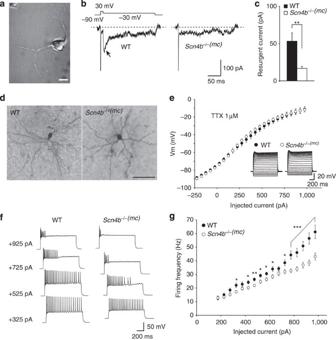Figure 8: Depletion of β4 decreased resurgent Na+current and compromised repetitive firing property in MSNs. (a) A photograph showing an isolated medium-sized neuron taken from the striatum. (b) Transient, persistent and resurgent Na+currents in a WT cell and aScn4b−/−(mc)cell. Tetrodotoxin-sensitive Na+currents were evoked by a 10-ms depolarization from −90 mV to +30 mV, followed by a 200-ms repolarization to −30 mV. Arrow shows the peak of the resurgent current. Transient Na+currents were truncated. (c) Resurgent Na+current was significantly reduced inScn4b−/−(mc)mice relative to their WT littermates. Data are presented as mean±s.e.m. (n=11 slices from 4 WT;n=22 slices from 5Scn4b−/−(mc)). **P<0.01, unpaired Student’st-test. (d) Each photograph shows a biocytin-filled and stained MSN in a brain slice taken from a WT orScn4b−/−(mc)mouse. (e) Composite current-voltage relationship for MSNs from WT andScn4b−/−(mc)mice recorded in the presence of tetrodotoxin (TTX 1 μM). Data are presented as mean±s.e.m. (n=15 slices from 2 mice per genotype).P>0.05, unpaired Student’st-test. (f) Spike discharge in response to current pulses of increasing intensity for a WT andScn4b−/−(mc)neuron. Note the strong reduction in the amplitude and frequency of spikes and the duration of repetitive firing for mutant compared with WT. (g) Average firing frequency was plotted as a function of step current injection. β4 is required for normal excitability in MSNs. Data are presented as mean±s.e.m. (775 pA,n=50 slices from WT;n=57 slices fromScn4b−/−(mc); 825 and 875 pA,n=50 slices from WT;n=57 slices fromScn4b−/−(mc); 925 and 975 pA,n=49 slices from WT;n=56 slices fromScn4b−/−(mc), the slices were prepared from 6 mice per genotype). *P<0.05, **P<0.01, and ***P<0.001, unpaired Student’st-test. Scale bars, 10 μm (a); 50 μm (d). Figure 8: Depletion of β4 decreased resurgent Na + current and compromised repetitive firing property in MSNs. ( a ) A photograph showing an isolated medium-sized neuron taken from the striatum. ( b ) Transient, persistent and resurgent Na + currents in a WT cell and a Scn4b −/−(mc) cell. Tetrodotoxin-sensitive Na + currents were evoked by a 10-ms depolarization from −90 mV to +30 mV, followed by a 200-ms repolarization to −30 mV. Arrow shows the peak of the resurgent current. Transient Na + currents were truncated. ( c ) Resurgent Na + current was significantly reduced in Scn4b −/−(mc) mice relative to their WT littermates. Data are presented as mean±s.e.m. ( n =11 slices from 4 WT; n =22 slices from 5 Scn4b −/−(mc) ). ** P <0.01, unpaired Student’s t -test. ( d ) Each photograph shows a biocytin-filled and stained MSN in a brain slice taken from a WT or Scn4b −/−(mc) mouse. ( e ) Composite current-voltage relationship for MSNs from WT and Scn4b −/−(mc) mice recorded in the presence of tetrodotoxin (TTX 1 μM). Data are presented as mean±s.e.m. ( n =15 slices from 2 mice per genotype). P >0.05, unpaired Student’s t -test. ( f ) Spike discharge in response to current pulses of increasing intensity for a WT and Scn4b −/−(mc) neuron. Note the strong reduction in the amplitude and frequency of spikes and the duration of repetitive firing for mutant compared with WT. ( g ) Average firing frequency was plotted as a function of step current injection. β4 is required for normal excitability in MSNs. Data are presented as mean±s.e.m. (775 pA, n =50 slices from WT; n =57 slices from Scn4b −/−(mc) ; 825 and 875 pA, n =50 slices from WT; n =57 slices from Scn4b −/−(mc) ; 925 and 975 pA, n =49 slices from WT; n =56 slices from Scn4b −/−(mc) , the slices were prepared from 6 mice per genotype). * P <0.05, ** P <0.01, and *** P <0.001, unpaired Student’s t -test. Scale bars, 10 μm ( a ); 50 μm ( d ). Full size image TTX-sensitive Na + currents were evoked by a 10-ms depolarization from −90 mV to +30 mV, followed by a 200-ms repolarization to −30 mV. The initial step depolarization to +30 mV evoked a transient Na + current ( I NaT ), which was followed by a persistent ( I NaP ) and I NaR at repolarization to −30 mV. The amplitude of I NaR was calculated as the peak current minus the amplitude of the current remaining at the end of the repolarizing pulse, the I NaP ( Fig. 8b ). I NaR in cells taken from WT mice was significantly larger than that in Scn4b −/−(mc) cells ( Fig. 8c and Table 1a , P <0.01). By contrast, there were no statistical differences in I NaT or I NaP between WT and Scn4b −/−(mc) mice ( Table 1b,c ). Thus, depletion of β4 significantly reduced the amplitude of I NaR in MSNs. Table 1 Electrophysiological results in WT and Scn4b −/−(mc) mice. Full size table Reduction of I NaR disrupts repetitive firing. We therefore tested whether depletion of β4 altered the electrophysiological properties of MSNs in whole-cell current clamp recordings in slice preparation. Experiments were performed in the presence of 2-amino-5-phosphonovaleric acid (APV, 50 μM), 6-cyano-7-nitroquinoxaline-2,3-dione (CNQX, 10 μM) and picrotoxin (PTX, 100 μM) to block glutamatergic and GABAergic synaptic transmission. Striatal MSNs showed a delayed spike firing in response to near-threshold depolarizing current pulses and a marked inward rectification to hyperpolarizing current pulses. Some of the recorded neurons were intracellularly injected with biocytin and stained to morphologically confirm their cell type at the end of the recording period ( Fig. 8d ). There was no discernible morphological difference between WT and Scn4b −/−(mc) mice. Likewise, no significant differences were found between the two in resting membrane potential ( Table 1d ), input resistance at −70 mV ( Table 1e ), half spike width ( Table 1f ) or rise time constant at −80 mV ( Table 1g ). The voltage-current (V-I) relationship recorded from −90 to −10 mV in the presence of TTX also revealed no differences between the two ( Fig. 8e ). Next, we compared repetitive firing properties of MSNs between WT and Scn4b −/−(mc) mice. To stimulate MSNs with certainty and high frequency, we used two strategies. First, we placed two tungsten or glass electrodes in the striatum, antidromically stimulated axon fibres with 50 pulses of 100-μs duration and a sufficiently small intensity of 0.2~1.0 mA at 100, 133 and 200 Hz and tested how many spikes were evoked in the recorded neurons by 50 electrical stimuli. No differences could be found between the two in this test ( Table 1h ). Second, we injected 20 current pulses of 1~3 ms duration and 1 nA into the cells examined at 100, 133 and 200 Hz and tested how many spikes were evoked. Although we found no statistical differences between the two in spike number ( Table 1i ), there was a significant difference in the frequency of action potentials spontaneously evoked by current injection of 1 s duration. We increased the injected current of 1 s duration from 25 pA up to 975 pA in 50-pA increments to compare average firing frequency between the two. Although rheobase for WT was equivalent to that for Scn4b −/−(mc) mice ( Table 1j ), average firing frequency in Scn4b −/−(mc) mice was significantly more decreased than that in WT when the injected current was more than 325 pA, except for 375 and 675 pA ( Fig. 8f,g , P <0.001 from 775 to 975 pA). Thus, it appears that depletion of β4 significantly decreases repetitive firing frequency in the face of constant depolarization. We next examined whether depletion of β4 altered conduction velocity in MSNs. First, action potentials were antidromically evoked in striatal cells by electrical stimulation with one or two electrodes placed in the striatum. The distances between the cells recorded and the electrodes were measured using photos taken after the experiments. The conduction velocities were estimated by the distances divided by the latencies of action potentials from stimulus artifacts. We found that the conduction velocities in both WT and Scn4b −/−(mc) mice were similar and not significantly different from each other ( Table 1k ). Second, we used sagittal slices obtained from Scn4b −/−(mc) mice crossed with Scn4b-Venus transgenic mice ( WT-Venus or Scn4b −/−(mc) -Venus mice) whose striatonigral pathways were visible under fluorescent microscope with Venus. Two electrodes were placed apart on the bright striatonigral pathways ( Fig. 9a ) and the inhibitory postsynaptic currents (eIPSCs) evoked by electrical stimulation were measured from the stimulus artefacts to the onset of eIPSCs from nigral neurons in whole-cell voltage-clamp mode ( Fig. 9b ). Stimulation electrodes and recording patch pipettes were positioned almost linearly, and the distances among them were measured to calculate the conduction velocities ( Fig. 9c ). Again, there were no significant differences in the conduction velocities between WT-Venus and Scn4b −/−(mc) -Venus mice ( Fig. 9d and Table 1l ). Estimated synaptic delays of eIPSCs in WT-Venus and Scn4b −/−(mc) -Venus mice were also similar ( Table 1m ). We also examined paired pulse ratios of eIPSCs and found a tendency to respond more vigorously to the second stimulus given 50 ms after the first stimulus in the nigral neurons of both types of mice, but no significant differences were found between the two ( Fig. 9e and Table 1n ). Failure rates significantly increased in Scn4b −/−(mc) -Venus mice compared with WT-Venus mice ( Fig. 9f,g and Table 1o ). 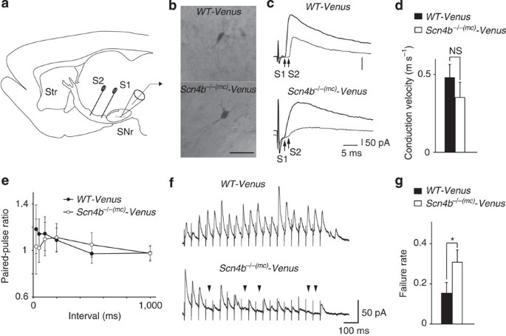Figure 9: Deletion of β4 increased failure rates of evoked IPSCs in nigral neurons. (a) Schema showing the recording configuration of nigral neurons in a sagittal slice (SNr=substantia nigra pars reticulata; Str=striatum). Two stimulating electrodes (S1, S2) were placed on the striatonigral pathways. (b) Photographs showing biocytin-filled and stained nigral neurons in a brain slice of aWT-Venusor aScn4b−/−(mc)-Venusmouse. Scale bar, 50 μm. (c) IPSCs evoked with two electrodes (S1, solid line; S2, dotted line) in nigral neurons of aWT-Venusor aScn4b−/−(mc)-Venusmouse. Arrows indicate onsets of the eIPSCs. (d) Summary of conduction velocities. Data are presented as mean±s.e.m. (n=10 slices fromWT-Venus;n=11 slices fromScn4b−/−(mc)-Venus, the slices were prepared from six mice per genotype). NS, not significant,P>0.05, unpaired Student’st-test. (e) Paired pulse ratio of eIPSCs. (n=17 slices fromWT-Venus;n=20 slices fromScn4b−/−(mc)-Venus, the slices were prepared from five mice per genotype).P>0.05, unpaired Student’st-test. (f) IPSCs evoked with repetitive stimulation (20 pulses, 20 Hz). Arrowheads indicate failures of the eIPSCs. Data are presented as mean±s.e.m. (g) Summary of the failure rates of the eIPSCs. Data are presented as mean±s.e.m. (n=16 slices fromWT-Venus;n=19 slices fromScn4b−/−(mc)-Venus, the slices were prepared from five mice per genotype). *P<0.05, unpaired Student’st-test. Figure 9: Deletion of β4 increased failure rates of evoked IPSCs in nigral neurons. ( a ) Schema showing the recording configuration of nigral neurons in a sagittal slice (SNr=substantia nigra pars reticulata; Str=striatum). Two stimulating electrodes (S1, S2) were placed on the striatonigral pathways. ( b ) Photographs showing biocytin-filled and stained nigral neurons in a brain slice of a WT-Venus or a Scn4b −/−(mc) -Venus mouse. Scale bar, 50 μm. ( c ) IPSCs evoked with two electrodes (S1, solid line; S2, dotted line) in nigral neurons of a WT-Venus or a Scn4b −/−(mc) -Venus mouse. Arrows indicate onsets of the eIPSCs. ( d ) Summary of conduction velocities. Data are presented as mean±s.e.m. ( n =10 slices from WT-Venus ; n =11 slices from Scn4b −/−(mc) -Venus , the slices were prepared from six mice per genotype). NS, not significant, P >0.05, unpaired Student’s t -test. ( e ) Paired pulse ratio of eIPSCs. ( n =17 slices from WT-Venus ; n =20 slices from Scn4b −/−(mc) -Venus , the slices were prepared from five mice per genotype). P >0.05, unpaired Student’s t -test. ( f ) IPSCs evoked with repetitive stimulation (20 pulses, 20 Hz). Arrowheads indicate failures of the eIPSCs. Data are presented as mean±s.e.m. ( g ) Summary of the failure rates of the eIPSCs. Data are presented as mean±s.e.m. ( n =16 slices from WT-Venus ; n =19 slices from Scn4b −/−(mc) -Venus , the slices were prepared from five mice per genotype). * P <0.05, unpaired Student’s t -test. Full size image In this study, we found atypical localization of β4 in striatal projection fibres, showing non-focal and diffuse β4 distribution along the axons. Those fibres lack nodes of Ranvier and immunoreactivity of MBP and NFH, and an EM study confirmed they are unmyelinated. Thus, the unique diffuse staining pattern of β4 (along with the lack of certain myelinated axonal markers) can positively define β4-bearing unmyelinated fibres. Several electron microscopic studies have reported D1R immunoreactivity in myelinated and unmyelinated axons around SNr [25] , [26] , [27] , and D2R-positive unmyelinated axons were detected in the striatum [28] and ventral pallidum [29] . These results suggest that striatal projection could include unmyelinated axons. However, due to methodological limitations of those EM studies, it was hard to determine the origin of axons and what portion of the striatal projection fibres contains unmyelinated fibres. We sought to clarify this point using Scn4b-Venus mice, which express Venus in MSNs and their projection fibres including the direct and indirect pathways. Venus expression completely colocalized with β4 diffuse staining, suggesting that virtually all β4-expressing projection fibres from striatum are unmylinated. Using PPE-GFP mice, we further confirmed that the indirect pathway is composed of unmyelinated fibres. These results demonstrate the existence of large bundles of unmyelinated projection fibres from the striatum. The role of unmyelinated fibres in the CNS is not well known. It has been thought that the mammalian CNS had abandoned unmyelinated nerve fibres in favour of myelinated fibres, as unmyelinated fibres are slow-conducting and energetically expensive [30] . However, the preservation of such long, large bundles of unmyelinated fibres as striatal projection fibres suggests potential beneficial effects in the circuit. A massive unmyelinated axonal arbor was reported in the nigrostriatal pathway [31] . We also examined myelination of this pathway by immunohistochemistry, suggesting this pathway could be unmyelinated or partly thin-myelinated ( Supplementary Fig. 5 ). So the main circuit (input and output) in the striatum could have slow conductance. This might be beneficial for motor control and reward processing by the basal ganglia. In the hippocampus, well-known unmyelinated fibres called mossy fibres originate from granular cells, which show adult neurogenesis; unmyelinated fibres might be beneficial because myelin is a main blocker to regeneration, although it is not known whether neurogenesis occurs in the striatum [32] . Another unique feature of unmyelinated fibres was recently discovered: vesicular release of glutamate from unmyelinated fibres in the corpus callosum, which are responsible for glutamatergic signalling with NG2 + glia [33] , [34] . Thus, unmyelinated fibres might mediate the release of neurotransmitters from the axonal surface. In this study, we found Nav1.2 diffusely localized on these axons, co-localizing with β4. Nav1.2 was previously reported to localize in the unmyelinated fibres of optic nerves, hippocampus and cerebellum [22] , [23] . We also confirmed diffuse Nav1.2 immunoreactivity on the mossy fibres of hippocampus and the parallel fibres of cerebellum (data not shown), suggesting Nav1.2 is diffusely distributed on unmyelinated fibres in CNS including striatal projection fibres. The striatal projection fibres are GABAergic and inhibitory, although many known unmyelinated fibres are glutamatergic and excitatory. Thus, the question arises whether β4 is also expressed in those unmyelinated glutamatergic axons. To examine this, we stained the corpus callosum with anti-mSCN4B-C and anti-Nav1.2. Diffuse β4 staining was not observed in the corpus callosum, but Nav1.2 was diffusely distributed in a portion of corpus callosum axons ( Supplementary Fig. 6a,b ). Thus, the results suggest that β4 is expressed in the GABAergic unmyelinated axons and Nav1.2 seems to be more generally expressed in unmyelinated axons, including those of corpus callosum. In the present study, we found elevated β4 dimer levels in striatonigral fibres. However, there were no overt changes evident in immunostaining and EM studies in the fascicles of striatal projection axons in Scn4b − / − mice. It is broadly accepted that β1 serves as a CAM [2] , [4] , [35] . During early postnatal development, β1 is expressed in the mouse forebrain as early as P1 (ref. 36 ), but β4 expression begins in the mouse brain between P1 and P7 ( Supplementary Fig. 7 ). These results give rise to the possibility that β4 might not contribute to pathfinding in early postnatal development, but may play an auxiliary role during later development. It has been proposed that the functions of IgCAMs on the basis of in vitro assay (for example, neurite outgrowth and cell migration) may not be affected in vivo when only one gene is ablated in a knockout mouse, because similar and overlapping functions of IgCAMs provide compensation. NrCAM-null mouse cerebellum showed no marked changes, but NrCAM and L1 double-knockout mice exhibited severe cerebellar folial defects and size reduction [37] . Thus, the effects of β4 ablation in vivo are possibly compensated by other IgCAMs members. On membrane depolarization, VGSCs first activate (open) and then inactivate (close), carrying the classic ‘transient’ inward Na + current ( I NaT ). In addition to this rapidly inactivating I NaT , VGSCs generate two distinct inward Na + currents in some neurons: a non-inactivating ‘persistent’ Na + current ( I NaP ) and a ‘resurgent’ Na + current ( I NaR ). I NaP is activated at sub-threshold potentials of about −60 to −50 mV and may facilitate bursts of neuronal discharges [38] . I NaR is also a transient current generated when action potential generation and channel inactivation ( I NaT ) is followed by membrane repolarization to voltages near −50 or −60 mV and has been implicated in repetitive action potential discharges of neurons [11] . To date, the most accepted mechanism to explain how I NaR is produced is an open-channel block by the cytoplasmic tail of an accessory subunit β4 of VGSC [9] , [10] . Grieco et al. [10] demonstrated that a free peptide containing the cytoplasmic tail of β4 restored the resurgent currents after enzymatic degradation of the endogenous open-channel blocker by trypsin and chymotrypsin in inside-out patches taken from cerebellar Purkinje neurons. Bant and Raman [9] confirmed their results by showing that the knockdown of Scn4b (elimination of β4) with its siRNA in cultured cerebellar granule neurons led to a loss of I NaR , a reduction of I NaP , a higher rheobase and a decrease in repetitive firing. We previously showed that MSNs of the striatum have β4, which is downregulated in HD model mice and in human patients [12] . Therefore, we predicted that the I NaR would be present in MSNs of WT mice but not in those of Scn4b -null mice. As expected, our electrophysiological analysis using dissociated putative MSNs revealed that the I NaR of MSNs was significantly reduced in the Scn4b -null mice compared with WT controls, whereas I NaT and I NaP of MSNs of the Scn4b -null and WT mice were not statistically different from each other. The next question is the physiological relevance of I NaR in MSNs. It has been proposed that the I NaR immediately after a spike may promote high-frequency spontaneous firing of neurons [2] , [39] , [40] , [41] , [42] , [43] . Our whole-cell current clamp recordings in brain slices showed that spontaneous firing during sustained depolarization in MSNs of Scn4b -null mice was significantly attenuated at injected currents of more than 325 pA compared with WT mice, whereas the relationship of membrane potential and injected current in MSNs was almost identical between Scn4b -null and WT mice. Thus, β4 considerably influences excitability of MSNs. β4 may enable MSNs to discharge significantly higher-frequency spikes for a long time when MSNs are in the Up-state of −71 to −40 mV in vivo , which is maintained by a barrage of synaptic excitation [44] . Furthermore, deletion of β4 increased failure rates of striatonigral inputs in response to 20-pulse stimulation at 20 Hz. The most general cause of the increased failure rate is reduction of release probability at the presynaptic terminal [45] . In our experiments, the paired pulse ratio was not significantly different between the mutant mice and the WT control mice, so an apparent change of release probability appears unlikely in this case. Another possible factor in transmission failure is collapse of spike propagation. Yang and Wang [46] demonstrated that spike propagation in axons of Purkinje cells is more reliable during application of anemone toxin II, which blocks inactivation of VGSC and enhances resurgent currents [46] , [47] . Although it remains to be studied whether I NaR directly regulates the failure rate, deletion of β4 could influence the spike propagation in striatonigral projections. Interestingly, in the tight unmyelinated axon bundle of the olfactory nerve, the ‘ephaptic’ interaction can lead to synchronized firing of independently stimulated axons [48] . In this regard, although we could not observe loosening of axon fasciculation in Scn4b -null mice, the depletion of β4 would be inconvenient for electrical interaction through the invisible extracellular space [49] . In any case, reduction of the number and frequency of spikes during the Up-state might somehow cause involuntary movements such as tremor-like movement observed in Scn4b -null mice and choreic movement in HD, which shows reduced β4 expression. In contrast, we found a slow conduction velocity of MSN axons of WT mice, which is compatible with a previous report [50] and with the fact that those axons are unmyelinated. The conduction velocity of MSN axons in Scn4b -null mice was not significantly different from that of WT mice, indicating that the densities of VGSCs along MSN axons and their diameters might be unaffected by deletion of β4. This was confirmed by examining the distribution of Nav1.2 in Scn4b −/−(mc) -Venus mouse. Nav1.2 is localized throughout the Venus-positive striatal projection fibres in WT-Venus mouse, and the similar distribution of Nav1.2 immunoreactivity was observed in Scn4b −/−(mc) -Venus mouse ( Supplementary Fig. 8 ). This result suggests that Nav1.2 localization was not affected by β4 ablation. VGSCs are key molecules of epilepsy and cardiac death [51] , [52] . β4 is expressed in both the brain and heart, and interacts with Nav1.5, which is the major α-subunit in heart cells [53] . It has been reported that SCN4B mutations are associated with cardiac death [53] , [54] , whereas SCN4B mutations related to epilepsy have not been identified. We observed sudden unexpected death in Scn4b -null mice without seizure, suggesting that β4 ablation might be related to a cardiac abnormality rather than epilepsy. In summary, we found atypical localization of β4 in the striatum, leading us to identify striatal projection fibres forming large unmyelinated inhibitory fibre bundles and to confirm that β4 functions as a physiological channel modulator in striatal MSNs. Antibodies Antibodies were listed in Supplementary Table 1 . Generation of anti-SCN4B antibodies Rat monoclonal anti-hSCN4B-C (7D7F10) antibody was generated against KLH-conjugated oligopeptides corresponding to the C-terminal region of human β4 (amino acids 209–228). Hybridoma supernatants were screened by ELISA, and then selected subclones were further analysed by western blot and immunohistochemistry. Conditioned media of a selected clone (7D7F10) were harvested from the stable hybridoma cultures, and antibody was purified using a HiTrap SP HP column (GE Healthcare) by Cell Engineering Corporation (Osaka, Japan). Rabbit polyclonal anti-mSCN4B-EC antibody was generated against recombinant protein corresponding to the extracellular region of mouse β4 (amino acid 30–160). Animals We generated three genetically modified mice. One is Scn4b-Venus transgenic mouse, which expresses the fluorescent marker Venus under the control of the 9-kb Scn4b promoter ( Fig. 3a ) (Details are described in Supplementary Methods ) and others are Scn4b -deficient mice with or without mCherry-V5-His and neomycin-resistant gene cassettes ( Fig. 6a ), which are described as Scn4b −/−(mc) and Scn4b −/− mice, respectively (Details are described in Supplementary Methods ). To visualize striatonigral projection fibres of the Scn4b deficient mice, Scn4b (mc) mutant mouse was crossed with Scn4b-Venus transgenic mouse. All experiments were carried out in accordance with the guidelines for Animal Care of the Riken Brain Science Institute. Both male and female mice were used for this study. Tissue preparation For in situ hybridization (ISH) and immunohistochemistry (IHC), mice were perfused with PBS followed by 4% paraformaldehyde (PFA) in PBS. To prepare frozen sections, brains were postfixed by 4% PFA in PBS overnight, immersed in 30% sucrose (wt/vol) in PBS, embedded in OCT compound, immediately frozen by solid CO 2 and stored at −80 °C. We cut 20-μm-thick sections with an HM 560 CryoStar Cryostat (Thermo Scientific) and 100-μm-thick sections were cut with a ROM380-CN sliding microtome (Yamato Kohki). To prepare paraffin sections, brains were postfixed, dehydrated and embedded in paraffin wax. Five- μm-thick sections were cut with an HM430 sliding microtome (Leica). ISH A cDNA fragment encoding Scn4b was obtained from IMAGE clone (IMAGE 1282676). cDNA fragments encoding Scn1b , Scn2b and Scn3b were amplified using KOD-plus polymerase (Toyobo) with specific primers anchored with appropriate restriction enzyme recognition sites ( Scn1b , Scn2b ) or SP6 promoter sequence ( Scn3b ). Amplified Scn1b and Scn2b cDNA were subcloned into pcDNA3.1/V5-His C vector (Invitrogen) and the sequences were confirmed by DNA sequencing. NotI-digested Scn1b , Scn2b and Scn4b , as well as amplified Scn3b , were used as templates to synthesize Digoxigenin-labelled cRNA probes. Those probes were prepared by MEGAscript T3 ( Scn4b ), T7 ( Scn1b and Scn2b ) or SP6 ( Scn3b ) Kit (Invitrogen) and DIG RNA Labelling Mix (Roche) according to the manufacturer’s instructions. Sections were incubated with PBS for 10 min, postfixed with 4% formalin/PBS for 5 min, acetylated with 0.25% acetic anhydride/0.1 M triethanolamine (pH 8.0) for 10 min and washed with PBS. The sections were incubated in a prehybridization solution (50% formamide, 5 × SSPE, 0.1% SDS, 1 mg Yeast tRNA (Roche)) for 2 h at 60 °C, and then hybridized with digoxigenin-labelled cRNA probe (1 ng μl −1 cRNA probe containing prehybridization solution) overnight at 60 °C. Next, sections were washed with 2 × SSC/50% formamide for 15 min at 50 °C two times and sequentially treated with RNase buffer (20 μg ml −1 RNase A (Sigma) containing 10 mM Tris–HCl, pH 8.0, 10 mM EDTA, 0.5 M NaCl) for 15 min at 37 °C; 2 × SSC for 15 min at 37 °C, two times; 0.2 × SSC for 15 min at 37 °C, two times. The sections were replaced in TBS and incubated with Blocking Regent (Roche) for 1 h, followed by alkaline phosphatase-conjugated anti-digoxigenin antibody, which was diluted with Solution B of Can Get Signal Immunostain (Toyobo) to enhance the signal, for 1 h. The sections were washed with TBST (0.05% TritonX-100) for 10 min, two times, and then treated with NTMT (0.1 M Tris-HCl (pH9.5)/0.1 M NaCl/0.05 M MgCl 2 /0.1% Tween 20) for 10 min. To visualize the signal, sections were developed with BCIP/NBT (Roche) diluted with NTMT/10% polyvinyl alcohol according to the manufacturer’s instruction for 2-3 days at 4 °C. IHC Autoclaved paraffin sections and 20-μm-thick frozen sections were incubated with blocking solution containing 5% skim milk in TBST, for 1 h. The sections were incubated with primary antibodies in TBST for overnight at 4 °C, followed by secondary antibodies. For diaminobenzidine (DAB) staining, sections were quenched 3% H 2 O 2 /methanol for 30 min before blocking, and incubated with VECTASTAIN Elite ABC Kit (Vector Laboratories) for 30 min after secondary antibody incubation. Then they were developed with substrate solution (0.1% DAB/0.015% peroxidase/0.05 M Tris–HCl (pH7.6)). Hundred- μm-thick frozen sections were stained by the following floating method. The sections were permeabilized with 0.2% TritonX-100 and incubated with blocking solution containing 2% BSA in TBST. The sections were transferred to primary antibody solution containing 2% BSA in TBST overnight at 4 °C, incubated with fluorescent secondary antibody solution containing 2% BSA in TBST for 3 h and then mounted with VECTASHIELD Mounting Medium (Vector Laboratories). Images were taken with a BIOREVO BZ-9000 (KEYENCE), TCS SP2 and SP5 confocal microscope (Leica), and we captured approximately the same area in each comparative sample. Combined staining of ISH ( Scn4b ) and IHC (anti-GFP) Procedures were combined for ISH and IHC with modification. Sections were pretreated and sequentially incubated with cRNA probe, RNase buffer, blocking regent and anti-digoxigenin antibody as ISH. To detect Venus immunoreactivity, sections were stained by anti-GFP (Roche), followed by Alexa Fluor 488 anti-mouse IgG. Fluorescent alkaline phosphatase activity was detected using HNPP Fluorescent Detection Set (Roche) according to the manufacturer’s instructions, and the sections were mounted with CC/Mount (Diagnostic BioSystems). Western blot Mouse brains or their subregions were rapidly isolated and homogenized with lysis buffer (20 mM Tris–HCl (pH 7.4), 150 mM NaCl, Complete Protease Inhibitor Cocktail Tablet, EDTA-free (Roche)). To remove debris and the nuclei fraction from the brain homogenates, they were centrifuged at 1,000 r.p.m. for 10 min at 4 °C. The supernatants were considered ‘brain lysate’. To purify the membrane fraction from the lysates, they were centrifuged at 40,000 r.p.m. for 20 min at 4 °C sequentially. Concentration of the protein samples was quantified by BCA assay (Thermo Fisher Scientific) followed by boiling with SDS sample buffer at 100 °C for 3 min. Protein samples were loaded onto 5–20% SDS-PAGE gels (ATTO), transferred onto PVDF membranes (Millipore) and incubated with primary antibodies overnight at 4 °C. After incubation with secondary antibodies, all blots were developed using Luminata Forte Western HRP substrate (Millipore). Images were taken by ImageQuant LAS 4000 (GE Healthcare) and band intensities on blots were quantified by NIH ImageJ. Full-size images of western blots are shown in Supplementary Fig. 10 . Tremor test A tremor test was carried out in 12-week-old male Scn4b mutant mice of each genotype. A mouse was placed in a semitransparent plastic box glued with an accelerometer (MVP-RF8-HC, MicroStone) at the bottom and moved freely. The box was suspended with thread. The motion of the mouse was recorded automatically for 1–5 min at a sampling rate of 1 kHz. Motion power percentage (MPP) [55] was calculated as (sum of amplitude at 20.5–40 Hz)/(sum of amplitude at 0–80 Hz) × 100 for each 1.024 s and averaged for every minute. Slice preparation and acute isolation of neurons The brain was removed from mice at P17-18, chilled, sliced (500-μm thick) coronally in ice-cold artificial cerebrospinal fluid (ACSF) containing the following components (in mM): 124 NaCl, 3 KCl, 1 NaH 2 PO 4 , 1.2 MgCl 2 , 2.4 CaCl 2 , 10 glucose, buffered to pH 7.4 with NaHCO 3 (26 mM), and saturated with 95% O 2 and 5% CO 2 where it was held for 1 h at room temperature. The slices were then placed in ACSF warmed to 31 °C, saturated with 95% O 2 and 5% CO 2 and containing pronase (0.17 mg ml −1 ) for 110 min. Enzyme digestion was terminated by transferring the slices to HEPES-buffered saline (HBS) maintained at 26 °C and containing the following (in mM): 150 NaCl, 5 KCl, 1 MgCl 2 , 10 glucose, 1 HEPES and 2 CaCl 2 , buffered to pH 7.4 with Tris–HCl (5 mM). The striatum was dissected from the slices and triturated for mechanical dissociation of neurons of the striatum and then placed in a recording chamber coated with poly- L -lysine for 15 min [56] . Phase-bright medium-sized neurons with a few sufficiently long neurites were chosen as MSNs in the striatum. Whole-cell voltage-clamp recordings in isolated neurons Whole-cell voltage-clamp recordings of Na + currents were performed in HBS at room temperature with an EPC9/2 amplifier and PULSE software (HEKA Elektronik, Lambrecht/Pfalz,; 5 kHz filtering, 50 kHz sampling), with infrared differential contrast visualization using a BX50WI microscope (Olympus, Dage-MTI). The internal solution contained the following (in mM): 110 CsCH 3 SO 3 , 11 CsCl, 2 MgCl 2 , 10 tetraethylammonium (TEA)-Cl, 10 HEPES, 4 Na 2 ATP, 0.3 NaGTP, 0.1 EGTA (pH 7.4 with CsOH). The external solutions used for recordings consisted of HBS containing (in mM) 10 TEA-Cl and 0.2 CdCl 2 with or without tetrodotoxin (TTX, 1 μM). Recordings were made first in HBS with TEA-Cl and CdCl 2 , and repeated in the same solutions but including TTX. TTX-sensitive Na + current was obtained by subtraction. Electrodes were pulled and fire-polished to yield resistance of 4–6 MΩ in the bath. For voltage-clamp recording, series resistance (8~35 MΩ; WT 14.8±1.8, n =17; Scn4b −/−(mc) 14.5±1.3, n =19) was compensated online by 50–70%. Liquid junction potential (~10 mV) was adjusted offline. Leak current subtraction was performed by a P/4 procedure. Whole-cell current-clamp recordings in slice preparation Coronal brain slices (250-μm thick) were obtained from mice at P30-58 as stated above and transferred to a recording chamber, which was continuously perfused with ACSF at a rate of 1–2 ml min −1 at 30 °C. Whole-cell current-clamp recordings (5 kHz filtering, 20 kHz sampling) were collected using patch pipettes (4~6 MΩ) containing the following (in mM): 129 K-gluconate, 11 KCl, 2 MgCl 2 , 10 HEPES, 4 Na 2 -ATP, 0.3 GTP and 0.5% biocytin (brought to pH 7.3 with KOH; osmolality, 280 mOsm). For current-clamp recording, series resistance (5~20 MΩ, WT 10.9±0.7, n =34, Scn4b −/−(mc) 11.6±0.6, n =32) was compensated online by 50–70%. Membrane potentials were not corrected for liquid junction potentials (~13 mV). Electron microscopy and pre-embedding immuno-EM For EM, mice were perfused with 2% PFA, 2.5% glutaraldehyde in 0.05 M sodium cacodylate (pH 7.4). Slices of striatum and substantia nigra were removed and postfixed overnight. Slices were fixed in 1% OsO4 in 0.05 M sodium cacodylate (pH 7.4) for 1 h, dehydrated in a graded series of ethanol and embedded in epoxy resin. Ultrathin (100 nm) coronal sections were prepared by ultramicrotome Leica EM UC6 (Leica) and stained 1% uranyl acetate solution for 15 min at 50 °C, followed by Lead stain solution (Sigma) for 10 min at room temperature. Stained sections were analysed with JEOL1200EX II (JEOL). For immune-EM, mice were perfused with 2% PFA, 0.5% glutaraldehyde in 0.05 M sodium cacodylate (pH 7.4). Coronal slices of striatum (200 μm-thick) were cut with a VT1000S vibrating blade microtome (Leica) and immersed 30% sucrose (wt/vol) in TBS. The slices were frozen with liquid nitrogen and thawed with TBS three times. The slices were incubated with TBS containing 0.1% H 2 O 2 for 1 h, followed by blocking solution (2% BSA in TBS) for 2 h. The slices were transferred to primary antibody solution (anti-mSCN4B-C, 1:3,000) containing 2% BSA in TBS overnight at 4 °C, incubated with biotinylated secondary antibody solution (1:500) containing 2% BSA in TBS for 3 h, and then incubated with VECTASTAIN Elite ABC Kit (Vector Laboratories) for 2 h, followed by DAB substrate solution (5 mg DAB/40 ml 0.05 M Tris–HCl (pH 7.4)/3 ul 0.3% H 2 O 2 ) for 20 min. The slices were fixed in 1% OsO4 solution, dehydrated in a graded series of ethanol and embedded in epoxy resin. Ultrathin (100–nm thick) coronal sections were stained using 1% uranyl acetate solution for 5 min at 50 °C, followed by Lead stain solution (Sigma) for 10 min at room temperature. Stained sections were analysed with JEOL1200EX II (JEOL). Statictics Sample sizes were determined on the basis of pilot experiments and previous experience from similar experiments. To examine whether the samples had the same variances, we first analysed them by F -test. We excluded an outlier sample calculated by Grubb’s test in Fig. 7b,c . All of the experiments were successfully repeated at least two times. Data are presented as means±s.e.m. and were analysed with the unpaired Student’s t -test, unpaired t -test with Welch’s correction or one-way ANOVA followed by Tukey’s post hoc test. * P <0.05, ** P <0.01, and *** P <0.001. A P -value of <0.05 was considered statistically significant. How to cite this article: Miyazaki, H. et al. Singular localization of sodium channel β4 subunit in unmyelinated fibres and its role in striatum. Nat. Commun. 5:5525 doi: 10.1038/ncomms6525 (2014).